Recovering three-dimensional shape around a corner using ultrafast time-of-flight imaging The recovery of objects obscured by scattering is an important goal in imaging and has been approached by exploiting, for example, coherence properties, ballistic photons or penetrating wavelengths. Common methods use scattered light transmitted through an occluding material, although these fail if the occluder is opaque. Light is scattered not only by transmission through objects, but also by multiple reflection from diffuse surfaces in a scene. This reflected light contains information about the scene that becomes mixed by the diffuse reflections before reaching the image sensor. This mixing is difficult to decode using traditional cameras. Here we report the combination of a time-of-flight technique and computational reconstruction algorithms to untangle image information mixed by diffuse reflection. We demonstrate a three-dimensional range camera able to look around a corner using diffusely reflected light that achieves sub-millimetre depth precision and centimetre lateral precision over 40 cm×40 cm×40 cm of hidden space. The light detected on an image sensor is composed of direct light, that travels directly from the light source to an object in the line of sight of the sensor, and indirect light that interacts with other parts of the scene before striking an object in the line of sight. Light from objects outside the line of sight reaches the sensor as indirect light, via multiple reflections (or bounces). In conventional imaging, it is difficult to exploit this non-line-of-sight light, if the reflections or bounces are diffuse. Line-of-sight time-of-flight information is commonly used in LIDAR (light detection and ranging) [1] and two dimensional gated viewing [2] to determine the object distance, or to reject unwanted scattered light. By considering only the early ballistic photons from a sample, these methods can image through turbid media or fog [3] . Other methods, like coherent LIDAR [4] , exploit the coherence of light to determine the time of flight. However, light that has undergone multiple diffuse reflections has diminished coherence. Recent methods in computer vision and inverse light transport study multiple diffuse reflections in free space. Dual photography [5] shows one can exploit scattered light to recover two-dimensional (2D) images of objects illuminated by a structured dynamic light source and hidden from the camera. Time-gated viewing using mirror reflections allows imaging around corners, for example, from a glass window [6] , [7] , [8] . Three bounce analysis of a time-of-flight camera can recover hidden 1–0–1 planar barcodes [9] , [10] but the technique assumes well-separated, isolated hidden patches with known correspondence between hidden patches and recorded pulses. Similar to these and other inverse light transport approaches [11] , we use a light source to illuminate one scene spot at a time and record the reflected light after its interaction with the scene. We demonstrate an incoherent ultrafast imaging technique to recover three-dimensional (3D) shapes of non-line-of-sight objects using this diffusely reflected light. We illuminate the scene with a short pulse and use the time of flight of returning light as a means to analyse direct and scattered light from the scene. We show that the extra temporal dimension of the observations under very high temporal sampling rates makes the hidden 3D structure observable. With a single or a few isolated hidden patches, pulses recorded after reflections are distinct and can be easily used to find 3D positions of the hidden patches. However, with multiple hidden scene points, the reflected pulses may overlap in both space and time when they arrive at the detector. The loss of correspondence between 3D scene points and their contributions to the detected pulse stream is the main technical challenge. We present a computational algorithm based on backprojection to invert this process. Our main contributions are twofold. We introduce the new problem of recovering the 3D structure of a hidden object and we show that the 3D information is retained in the temporal dimension after multi-bounce interactions between visible and occluded parts. We also present an experimental realization of the ability to recover the 3D structure of a hidden object, thereby demonstrating a 3D range camera able to look around a corner. The ability to record 3D shapes beyond the line of sight can potentially be applied in industrial inspection, endoscopy, disaster relief scenarios, or more generally, in situations where direct imaging of a scene is impossible. Imaging process The experimental set-up is shown in Fig. 1 . Our scene consists of a 40-cm high and 25-cm wide wall referred to as the diffuser wall. We use an ultrafast laser and a streak camera and both are directed at this wall. As a time reference, we also direct an attenuated portion of the laser beam into the field of view of the streak camera ( Fig. 2 ). The target object is hidden in the scene (mannequin in Fig. 1 ), so that direct light paths between the object and the laser or the camera are blocked. Our goal is to produce 3D range data of the target object. 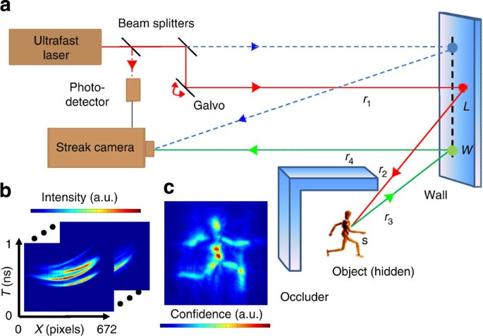Figure 1: Experimental set-up. (a) The capture process: we capture a series of images by sequentially illuminating a single spot on the wall with a pulsed laser and recording an image of the dashed line segment on the wall with a streak camera. The laser pulse travels a distancer1to strike the wall at a pointL; some of the diffusely scattered light strikes the hidden object (for example atsafter travelling a distancer2), returns to the wall (for example atw, after travelling overr3) and is collected by the camera after travelling the final distancer4fromwto the camera centre of projection. The position of the laser beam on the wall is changed by a set of galvanometer-actuated mirrors. (b) An example of streak images sequentially collected. Intensities are normalized against a calibration signal. Red corresponds to the maximum, blue to the minimum intensities. (c) The 2D projected view of the 3D shape of the hidden object, as recovered by the reconstruction algorithm. Here the same colour map corresponds to backprojected filtered intensities or confidence values of finding an object surface at the corresponding voxel. Figure 1: Experimental set-up. ( a ) The capture process: we capture a series of images by sequentially illuminating a single spot on the wall with a pulsed laser and recording an image of the dashed line segment on the wall with a streak camera. The laser pulse travels a distance r 1 to strike the wall at a point L ; some of the diffusely scattered light strikes the hidden object (for example at s after travelling a distance r 2 ), returns to the wall (for example at w , after travelling over r 3 ) and is collected by the camera after travelling the final distance r 4 from w to the camera centre of projection. The position of the laser beam on the wall is changed by a set of galvanometer-actuated mirrors. ( b ) An example of streak images sequentially collected. Intensities are normalized against a calibration signal. Red corresponds to the maximum, blue to the minimum intensities. ( c ) The 2D projected view of the 3D shape of the hidden object, as recovered by the reconstruction algorithm. Here the same colour map corresponds to backprojected filtered intensities or confidence values of finding an object surface at the corresponding voxel. 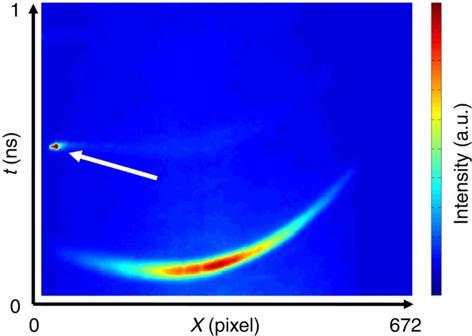Figure 2: Streak image with calibration spot. The calibration spot in a streak image (highlighted with an arrow). The calibration spot is created by an attenuated beam split off the laser beam that strikes the wall in the field of view of the camera. It allows monitoring of the long-term stability of the system and calibration for drifts in timing synchronization. Full size image Figure 2: Streak image with calibration spot. The calibration spot in a streak image (highlighted with an arrow). The calibration spot is created by an attenuated beam split off the laser beam that strikes the wall in the field of view of the camera. It allows monitoring of the long-term stability of the system and calibration for drifts in timing synchronization. Full size image The streak camera records a streak image with one spatial dimension and one temporal dimension. We focus the camera on the dashed line segment on the diffuser wall shown in Fig. 1a . We arrange the scanning laser to hit spots on the wall above or below this line segment so that single bounce light does not enter the camera. Though the target object is occluded, light from the laser beam is diffusely reflected by the wall, reaches the target object, is reflected by multiple surface patches, and returns back to the diffuser wall, where it is reflected again and captured by the camera. In a traditional camera, this image would contain little or no information about the occluded target object ( Supplementary Figs S5 and S6 ; Supplementary Methods ). In our experimental set-up, the laser emits 50-fs long pulses. The camera digitizes information in time intervals of 2 ps. We assume the geometry of the directly visible part of the set-up is known. Hence, the only unknown distances in the path of the laser pulses are those from the diffuser wall to the different points on the occluded target object and back (paths r 2 and r 3 in Fig. 1 ). The 3D geometry of the occluded target is thus encoded in the streak images acquired by the camera and decoded using our reconstruction algorithm. The recorded streak images lack correspondence information, that is, we do not know which pulses received by the camera came from which surface point on the target object. Hence, a straightforward triangulation or trilateration to determine the hidden geometry is not possible. Consider a simple scenario with a small hidden patch as illustrated in Fig. 3a . It provides intuition on how the geometry and location of the target object are encoded in the streak images. The reflected spherical pulse propagating from the hidden patch arrives at the points on the diffuser wall with different time delays and creates a hyperbolic curve in the space-time streak image. We scan and successively change the position of the laser spot on the diffuser wall. The shape and position of the recorded hyperbolic curve varies accordingly. Each pixel in a streak image corresponds to a finite area on the wall and a 2-ps time interval, a discretized space-time bin. However, the effective time resolution of the system is 15 ps owing to a finite temporal-point spread function of the camera. The detailed description of image formation is included in the Supplementary Methods . 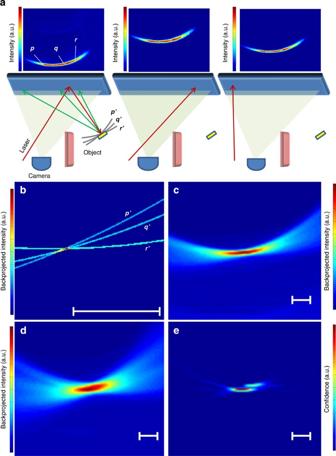Figure 3: Reconstruction algorithm. An illustrative example of geometric reconstruction using streak camera images. (a) Data capture. The object to be recovered consists of a 2 cm×2 cm size square white patch beyond the line of sight (that is, hidden). The patch is mounted in the scene and data is collected for different laser positions. The captured streak images corresponding to three different laser positions are displayed in the top row. Shapes and timings of the recorded response vary with laser positions and encode the position and shape of the hidden patch. (b) Contributing voxels in Cartesian space. For recovery of hidden position, consider the choices of contributing locations. The possible locations in Cartesian space that could have contributed intensity to the streak image pixelsp,q,rare the ellipsesp′,q′,r′ (ellipsoids in 3D). For illustration, these three ellipse sections are also shown in (a) bottom left in Cartesian coordinates. If there is a single world point contributing intensity to all 3 pixels, the corresponding ellipses intersect, as is the case here. The white bar corresponds to 2 cm in all sub-figures. (c) Backprojection and heatmap. We use a backprojection algorithm that finds overlayed ellipses corresponding to all pixels, Here we show summation of elliptical curves from all pixels in the first streak image. (d) Backprojection using all pixels in a set of 59 streak images. (e) Filtering. After filtering with a second derivative, the patch location and 2-cm lateral size are recovered. Figure 3: Reconstruction algorithm. An illustrative example of geometric reconstruction using streak camera images. ( a ) Data capture. The object to be recovered consists of a 2 cm×2 cm size square white patch beyond the line of sight (that is, hidden). The patch is mounted in the scene and data is collected for different laser positions. The captured streak images corresponding to three different laser positions are displayed in the top row. Shapes and timings of the recorded response vary with laser positions and encode the position and shape of the hidden patch. ( b ) Contributing voxels in Cartesian space. For recovery of hidden position, consider the choices of contributing locations. The possible locations in Cartesian space that could have contributed intensity to the streak image pixels p , q , r are the ellipses p ′, q ′, r ′ (ellipsoids in 3D). For illustration, these three ellipse sections are also shown in ( a ) bottom left in Cartesian coordinates. If there is a single world point contributing intensity to all 3 pixels, the corresponding ellipses intersect, as is the case here. The white bar corresponds to 2 cm in all sub-figures. ( c ) Backprojection and heatmap. We use a backprojection algorithm that finds overlayed ellipses corresponding to all pixels, Here we show summation of elliptical curves from all pixels in the first streak image. ( d ) Backprojection using all pixels in a set of 59 streak images. ( e ) Filtering. After filtering with a second derivative, the patch location and 2-cm lateral size are recovered. Full size image The inverse process to recover the position of the small hidden patch from the streak images is illustrated in Fig. 3b–e . Consider three pixels p , q and r in the streak image at which non-zero light intensity is measured ( Fig. 3a ). The possible locations in the world that could have contributed to a given pixel lie on an ellipsoid in Cartesian space (see also Supplementary Fig. S1 ). The foci of this ellipsoid are the laser spot on the diffuser wall and the point on the wall observed by that pixel. For illustration, we draw only a 2D slice of the ellipsoid, that is, an ellipse, in Fig. 3b . The individual ellipses from each of the three pixels p , q and r intersect at a single point. In the absence of noise, the intersection of three ellipses uniquely determines the location of the hidden surface patch that contributed intensity to the three camera pixels. In practice, we lack correspondence, that is, we do not know whether or not light detected at two pixels came from the same 3D surface point. Therefore, we discretize the Cartesian space into voxels and compute the likelihood of the voxel being on a hidden surface. For each voxel, we determine all streak image pixels that could potentially have received contributions of this voxel based on the time-of-flight r 1 + r 2 + r 3 + r 4 and sum up the measured intensity values in these pixels. In effect, we let each pixel vote for all points on the corresponding ellipsoid. The signal energy contributed by each pixel is amplified by a factor to compensate for the distance attenuation. If the distance attenuation factor were not accounted for, the scene points that are far away from the wall would be attenuated by a factor of ( r 2 r 3 ) 2 and would be lost during the reconstruction. Therefore, we amplify the contribution of each pixel to a particular voxel by a factor of ( r 2 r 3 ) α before backprojection. Reconstruction quality depends weakly on the value of α . We experimented with various values of α and found that α =1 is a good choice for reduced computation time. This process of computing likelihood by summing up weighted intensities is called backprojection [12] . We call the resulting 3D scalar function on voxels a heatmap. The summation of weighted intensities from all pixels in a single-streak image creates an approximate heatmap for the target patch ( Fig. 3c ). Repeating the process for many laser positions on the diffuser wall, and using pixels from the corresponding streak images provides a better approximation ( Fig. 3d and Supplementary Fig. S2 ). In practice, we use ∼ 60 laser positions. Traditional backprojection requires a high-pass filtering step. We use the second derivative of the data along the z direction of the voxel grid and approximately perpendicular to the wall as an effective filter and recover the hidden surface patch in Fig. 3e . Because values at the voxels in the heatmap are the result of summing a large number of streak image pixels, the heatmap contains low noise and the noise amplification associated with a second-derivative filter is acceptable. Algorithm The first step of our imaging algorithm is data acquisition. We sequentially illuminate a single spot on the diffuser wall with a pulsed laser and record an image of the line segment of the wall with a streak camera. Then, we estimate an oriented bounding box for the working volume to set up a voxel grid in Cartesian space (see Methods ). In the backprojection, for each voxel, we record the summation of weighted intensities of all streak image pixels that could potentially have received contributions of this voxel based on the time of flight. We store the resulting 3D heatmap of voxels. The backprojection is followed by filtering. We compute a second derivative of the heatmap along the direction of the voxel grid facing away from the wall. In an optional post processing step, we compute a confidence value for each voxel by computing local contrast with respect to the voxel neighbourhood in the filtered heatmap. To compute contrast, we divide each voxel heatmap value by the maximum in the local neighbourhood. For better visualization, we apply a soft threshold on the voxel confidence value. We estimate the oriented bounding box of the object in the second step by running the above algorithm at low spatial target resolution and with down-sampled input data. Details of the reconstruction process and the algorithm can be found in the Methods as well as in the Supplementary Methods . Reconstructions We show results of the 3D reconstruction for multipart objects in Figs 4 and 5 . The mannequin in Fig. 4 contains nonplanar surfaces with variations in depth and occlusions. We accurately recover all major geometrical features of the object. 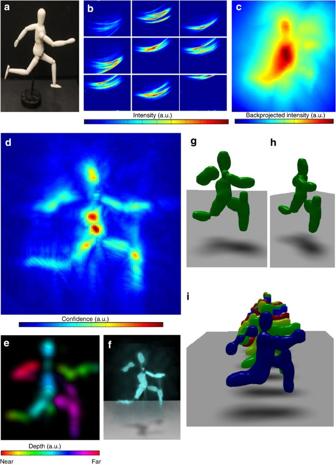Figure 4: Complex object reconstruction. (a) Photo of the object. The mannequin is∼20 cm tall and is placed about 25 cm from the diffuser wall. (b) Nine of the sixty raw streak images. (c) Heatmap. Visualization of the heatmap after backprojection. The maximum value along thezdirection for eachx–ycoordinate in Cartesian space. The hidden shape is barely discernible. (d) Filtering. The second derivative of the heatmap along depth (z) projected on thex–yplane reveals the hidden shape contour. (e) Depth map. Colour-encoded depth (distance from the diffuser wall) shows the left leg and right arm closer in depth compared with the torso and other leg and arm. (f) Confidence map. A rendered point cloud of confidence values after soft threshold. Images (g,h) show the object from different viewpoints after application of a volumetric blurring filter. (i) The stop-motion animation frames from multiple poses to demonstrate reproducability. SeeSupplementary Movie 1for an animation. Shadows and the ground plane in images (f–i) have been added to aid visualization. Figure 4i shows the reconstruction of the same object in slightly different poses to demonstrate the reproducibility and stability of the method as well as the consistency in the captured data. The sporadic inaccuracies in the reconstruction are consistent across poses and are confined to the same 3D locations. The stop-motion animation in Supplementary Movie 1 shows the local nature of the missing or phantom voxels more clearly; another stop motion reconstruction is shown in Supplementary Fig. S4 . Hence, the persistent inaccuracies are not due to signal noise or random measurement errors. This is promising as the voxel confidence errors are primarily due to limitations in the reconstruction algorithm and instrument calibration. These limitations can be overcome with more sophistication. Our current method is limited to diffuse reflection from near-Lambertian opaque surfaces. Parts of the object that are occluded from the diffuser wall or facing away from it are not reconstructed. Figure 4: Complex object reconstruction. ( a ) Photo of the object. The mannequin is ∼ 20 cm tall and is placed about 25 cm from the diffuser wall. ( b ) Nine of the sixty raw streak images. ( c ) Heatmap. Visualization of the heatmap after backprojection. The maximum value along the z direction for each x – y coordinate in Cartesian space. The hidden shape is barely discernible. ( d ) Filtering. The second derivative of the heatmap along depth ( z ) projected on the x – y plane reveals the hidden shape contour. ( e ) Depth map. Colour-encoded depth (distance from the diffuser wall) shows the left leg and right arm closer in depth compared with the torso and other leg and arm. ( f ) Confidence map. A rendered point cloud of confidence values after soft threshold. Images ( g , h ) show the object from different viewpoints after application of a volumetric blurring filter. ( i ) The stop-motion animation frames from multiple poses to demonstrate reproducability. See Supplementary Movie 1 for an animation. Shadows and the ground plane in images ( f – i ) have been added to aid visualization. 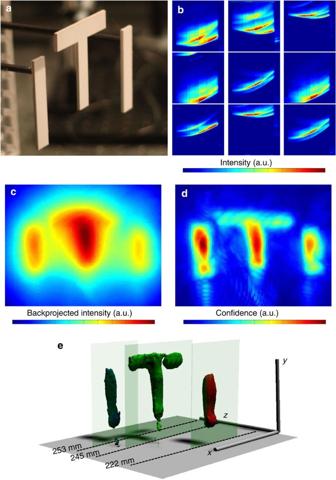Figure 5: Depth in reconstructions. Demonstration of the depth and lateral resolution. (a) The hidden objects to be recovered are three letters, I, T, I at varying depths. The 'I' is 1.5 cm wide and all letters are 8.2 cm high. (b) 9 of 60 images collected by the streak camera. (c) Projection of the heatmap created by the back projection algorithm, on thex–yplane. (d) Filtering after computing second derivative along depth (z). The colour in these images represents the confidence of finding an object at the pixel position. (e) A rendering of the reconstructed 3D shape. Depth is colour coded and semi-transparent planes are inserted to indicate the ground truth. The depth axis is scaled to aid visualization of the depth resolution. Full size image Figure 5: Depth in reconstructions. Demonstration of the depth and lateral resolution. ( a ) The hidden objects to be recovered are three letters, I, T, I at varying depths. The 'I' is 1.5 cm wide and all letters are 8.2 cm high. ( b ) 9 of 60 images collected by the streak camera. ( c ) Projection of the heatmap created by the back projection algorithm, on the x – y plane. ( d ) Filtering after computing second derivative along depth ( z ). The colour in these images represents the confidence of finding an object at the pixel position. ( e ) A rendering of the reconstructed 3D shape. Depth is colour coded and semi-transparent planes are inserted to indicate the ground truth. The depth axis is scaled to aid visualization of the depth resolution. Full size image Figure 5 shows a reconstruction of multiple planar objects at different unknown depths. The object planes and boundaries are reproduced accurately to demonstrate depth and lateral resolution. For further investigation of resolution see Supplementary Figs S7 and S8 . The reconstruction is affected by several factors such as calibration, sensor noise, scene size and time resolution. Below, we consider them individually. The sources of calibration errors are lens distortions on the streak camera that lead to a warping of the collected streak image, measurement inaccuracies in the visible geometry, and measurement inaccuracies of the centre of projection of the camera and the origin of the laser. For larger scenes, the impact of static calibration errors would be reduced. The sensor introduces intensity noise and timing uncertainty, that is, jitter. The reconstruction of 3D shapes is more dependent on the accuracy of the time of arrival than the signal-to-noise ratio (SNR) in received intensity. Jitter correction, as described in the Methods, is essential, but does not remove all uncertainties. Improving the SNR is desirable because it yields faster capture times. Similar to many commercial systems, for example, LIDAR, the SNR could be significantly improved by using an amplified laser with more energetic pulses and a repetition rate in the kilohertz range and a triggered camera. The overall light power would not change, but fewer measurements for light collection could significantly reduce signal independent noise such as background and shot noise. We could increase the scale of the system for larger distances and bigger target objects. By using a longer pulse, with proportionally reduced target resolution and increased aperture size, one could build systems without any change in the ratio of received and emitted energy, that is, the link budget. When the distance r 2 between diffuser wall and the hidden object ( Fig. 1 ) is increased without increasing the size of the object, the signal strength drops dramatically ( ∝ 1/( r 2 r 3 ) 2 ) and the size of the hidden scene is therefore limited. A configuration where laser and camera are very far from the rest of the scene is, however, plausible. A loss in received energy can be reduced in two ways. The laser beam can be kept collimated over relatively long distances and the aperture size of the camera can be increased to counterbalance a larger distance between camera and diffuser wall. The timing resolution, along with spatial diversity in the positions of spots illuminated and viewed by the laser, and the camera affects the resolution of 3D reconstructions. Extra factors include the position of the voxel in Cartesian space and the overall scene complexity. The performance evaluation subsection of the Supplementary Methods describes depth and lateral resolution. In our system, translation along the direction perpendicular to the diffuser wall can be resolved with a resolution of 400 μm—better than the full width half maximum time resolution of the imaging system. Lateral resolution in a plane parallel to the wall is lower and is limited to 0.5–1 cm depending on proximity to the wall. This paper's goals are twofold: to introduce the new challenging problem of recovering the 3D shape of a hidden object and to demonstrate the results using a novel co-design of an electro-optic hardware platform and a reconstruction algorithm. Designing and implementing a prototype for a specific application will provide further, more specific data about the performance of our approach in real-world scenarios. We have demonstrated the 3D imaging of a nontrivial hidden 3D geometry from scattered light in free space. We compensate for the loss of information in the spatial light distribution caused by the scattering process by capturing ultrafast time-of-flight information. Our reconstruction method assumes that light is only reflected once by a discrete surface on the hidden object without inter-reflections within the object and without subsurface scattering. We further assume that light travels in a straight line between reflections. Light that does not follow these assumptions will appear as time-delayed background in our heatmap and will complicate, but not necessarily prevent, reconstruction. The application of imaging beyond the line of sight is of interest for sensing in hazardous environments, such as inside machinery with moving parts, for monitoring highly contaminated areas such as the sites of chemical or radioactive leaks where even robots cannot operate or need to be discarded after use [13] . Disaster response and search and rescue planning, as well as autonomous robot navigation, can benefit from the ability to obtain complete information about the scene quickly [14] , [15] . A promising theoretical direction is in inference and inversion techniques that exploit scene priors, sparsity, rank, meaningful transforms, and achieve bounded approximations. Adaptive sampling can decide the next-best laser direction based on a current estimate of the 3D shape. Further analysis will include coded sampling using compressive techniques and noise models for SNR and effective bandwidth. Our current demonstration assumes friendly reflectance and planarity of the diffuse wall. The reconstruction of an image from diffusely scattered light is of interest in a variety of fields. Change in spatial light distribution due to the propagation through a turbid medium is in principle reversible [16] and allows imaging through turbid media via computational imaging techniques [17] , [18] , [19] . Careful modulation of light can shape or focus pulses in space and time inside a scattering medium [20] , [21] . Images of objects behind a diffuse screen, such as a shower curtain, can be recovered by exploiting the spatial frequency domain properties of direct and global components of scattered light in free space [22] . Our treatment of scattering is different but could be combined with many of these approaches. In the future, emerging integrated solid-state lasers, new sensors and nonlinear optics should provide practical and more sensitive imaging devices. Beyond 3D shape, new techniques should allow us to recover reflectance, refraction and scattering properties and achieve wavelength-resolved spectroscopy beyond the line of sight. The formulation could also be extended to shorter wavelengths (for example, X-rays) or to ultrasound and sonar frequencies. The new goal of hidden 3D shape recovery may inspire new research in the design of future ultrafast imaging systems and novel algorithms for hidden scene reconstruction. Capture set-up The light source is a Kerr lens mode-locked Ti:sapphire laser. It delivers pulses of about 50 fs length at a repetition rate of 75 MHz. Dispersion in the optical path of the pulse does not stretch the pulse beyond the resolution of the camera of 2 ps and therefore can be neglected. The laser wavelength is centred at 795 nm. The main laser beam is focused on the diffuser wall with a 1-m focal length lens. The spot created on the wall is about 1 mm in diameter and is scanned across the diffuser wall through a system of two galvanometer-actuated mirrors. A small portion of the laser beam is split off with a glass plate and is used to synchronize the laser and streak camera as shown in Fig. 1 . The diffuser wall is placed 62 cm from the camera. The mannequin object ( Fig. 4 ) is placed at a distance of about 25 cm to the wall, the letters ( Fig. 5 ) are placed at 22.2–25.3 cm. For time-jitter correction, another portion of the beam is split off, attenuated and directed at the wall as the calibration spot. The calibration spot is in the direct field of view of the camera and can be seen in Fig. 2 . The calibration spot serves as a time and intensity reference to compensate for drifts in the synchronization between laser and camera as well as changes in laser-output power. It also helps in detecting occasional shifts in the laser direction due to, for example, beam pointing instabilities in the laser. If a positional shift is detected, the data is discarded and the system is re-calibrated. The streak camera's photocathode tube, much like an oscilloscope, has time decayed burn out and local gain variations. We use a reference background photo to divide and compensate. The camera is a Hamamatsu C5680 streak camera that captures one spatial dimension, that is, a line segment in the scene, with an effective time resolution of 15 ps and a quantum efficiency of about 10%. The position and viewing direction of the camera are fixed. The diffuser wall is covered with Edmund Optics NT83 diffuse white paint. Reconstruction technique We use a set of Matlab routines to implement the backprojection-based reconstruction. Geometry information about the visible part of the scene, namely diffuser wall, could be collected using our time-of-flight system. Reconstructing 3D geometry of a visible scene using time-of-flight data is well known [2] . We omit this step and concentrate on the reconstruction of the hidden geometry. We use a FARO Gauge digitizer arm to measure the geometry of the visible scene and also to gather data about a sparse set of points on hidden objects for comparative verification. The digitizer arm data is used as ground truth for later independent verification of the position and shape of hidden objects as shown via transparent planes in Fig. 4e . After calibration, we treat the camera and laser as a rigid pair with known intrinsic and extrinsic parameters [23] . We estimate the oriented bounding box around the hidden object using a lower resolution reconstruction. We reduce the spatial resolution to 8 mm per voxel, and downsample the input data by a factor of 40. We can scan a 40 cm×40 cm×40 cm volume spanning the space in front of the wall in 2–4 s to determine the bounding box of a region of interest. The finer voxel grid resolution is 1.7 mm in each dimension. We can use the coarse reconstruction obtained to set up a finer grid within this bounding box. Alternatively, we can set an optimized bounding box from the collected ground truth. To minimize reconstruction time, we used this second method in most of the published reconstructions. We confirmed that apart from the reconstruction time and digitization artefacts, both methods produce the same results. We compute the principal axis of this low-resolution approximation, and orient the fine voxel grid with these axes. In the post-processing step, we use a common approach to improve the surface visualization. We estimate the local contrast and apply a soft threshold. The confidence value for a voxel is V ′=tanh(20( V − V 0 )) V / m loc , where V is the original voxel value in filtered heatmap and m loc is a local maximum computed in a 20×20×20 voxel sliding window around the voxel under consideration. Division by m loc normalizes for local contrast. The value V 0 is a global threshold and set to 0.3 times the global maximum of the filtered heatmap. The tanh function achieves a soft threshold. System SNR The laser emits a pulse every 13.3 ns (75 MHz) and consequently the reflected signal repeats at the same rate. We average 7.5 million such 13.3 ns windows in a 100-ms exposure time on our streak tube readout camera. We add 50–200 such images to minimize noise from the readout camera. The light returned from a single hidden patch is attenuated in the second, third and fourth path segments. In our set-ups, this attenuation factor is 10 −8 . Attenuation in the fourth path segment can be partially counteracted by increasing the camera aperture. Choice of laser positions on the wall Recall that we direct the laser to various positions on the diffuser wall and capture one streak image for each position. The position of a hidden point s ( Fig. 1 ) is determined with highest confidence along the normal N to an ellipsoid through s with foci at the laser spot, L , and the wall point, w . Large angular diversity through a wide range of angles for N for all such pairs to create baselines is important. N is the angle bisector of ∠ Lsw . The location and spacing of the laser positions on the wall can have a big impact on reconstruction performance. To obtain good results, one should choose the laser positions so as to provide good angular diversity. We use 60 laser positions in 3–5 lines perpendicular to the line on the wall observed by our one-dimensional streak camera. This configuration yielded significantly better results than putting the laser positions on few lines parallel to the camera line. Scaling the system Scaling up the distances in the scene is challenging because higher resolution and larger distances lead to disproportionately less light being transferred through the scene. A less challenging task may be to scale the entire experiment including the hidden object, the pulse length, the diffuser wall and the camera aperture. The reduction in resolution to be expected in this scaling should be equal to the increase in size of the hidden object. To understand this, consider a hidden square patch in the scene. To resolve it, we require discernible light to be reflected back from that patch after reflections or bounces off other patches. Excluding the collimated laser beam, there are three paths, as described earlier. For each path, light is attenuated by approximately d 2 /(2 πr 2 ), where r is the distance between the source and the destination patch and d is the side length of the destination patch. For the fourth segment, the destination patch is the camera aperture and d denotes the size of this aperture. If r and d are scaled together for any path, the contributed energy from the source patch to the destination patch does not change. This may allow us to scale the overall system to larger scenes without a prohibitively drastic change in performance. However, increasing the aperture size is only possible to a certain extent. Non-Lambertian surfaces Our reconstruction method is well-suited for Lambertian reflectance of surfaces. Our method is also robust for near-Lambertian surfaces, for example, surfaces with a large diffuse component, and they are implicitly handled in our current reconstruction algorithm. The surface reflectance profile only affects the relative weight of the backprojection ellipses and not their shapes. The shape is dictated by the time-of-flight, which is independent of the reflectance distribution. Surfaces that are highly specular, retroreflective or have a low reflectance make the hidden shape reconstruction challenging. Highly specular, mirror-like and retroreflective surfaces limit the regions illuminated by the subsequent bounces and may not reflect enough energy back to the camera. They also could cause dynamic range problems. Subsurface scattering or extra inter-reflections extend the fall time in reflected time profile of a pulse. But the onset due to reflection from the first surface is maintained in the time profile and hence the time delayed reflections appear as background noise in our reconstruction. Absorbing low-reflectance black materials reduce the SNR but the effect is minor compared with the squared attenuation over distances. Although near-Lambertian surfaces are very common in the proposed application areas, reconstruction in the presence of varying reflectance materials is an interesting future research topic. How to cite this article: Velten, A. et al . Recovering three-dimensional shape around a corner using ultrafast time-of-flight imaging. Nat. Commun. 3:745 doi: 10.1038/ncomms1747 (2012).